Structural isomerism in gold nanoparticles revealed by X-ray crystallography Revealing structural isomerism in nanoparticles using single-crystal X-ray crystallography remains a largely unresolved task, although it has been theoretically predicted with some experimental clues. Here we report a pair of structural isomers, Au 38T and Au 38Q , as evidenced using electrospray ionization mass spectrometry, X-ray photoelectron spectroscopy, thermogravimetric analysis and indisputable single-crystal X-ray crystallography. The two isomers show different optical and catalytic properties, and differences in stability. In addition, the less stable Au 38T can be irreversibly transformed to the more stable Au 38Q at 50 °C in toluene. This work may represent an important advance in revealing structural isomerism at the nanoscale. Structural isomerism in organic molecules is a common occurrence due to the bonding diversity of carbon. However, for nanoscale or even larger scale materials, experimental observation of structural isomerism has been largely impeded by the challenge of unravelling the intrinsic structure at the atomic level [1] . Nevertheless, theoretical and experimental efforts [2] , [3] , [4] , [5] , [6] , [7] , [8] in searching for structural isomerism in such materials continue, because such a finding would provide precise and insightful structure–property correlations and meaningful guidance for designing and synthesizing unique functional materials. The recently developed ultrasmall, thiolated metal nanoparticles (also called nanoclusters) provide opportunities for investigating structural isomerism, as they can now be controlled with atomic precision [9] , [10] , [11] , [12] , [13] , [14] , [15] , [16] , [17] , [18] , [19] , [20] and their structures can be resolved by single-crystal X-ray crystallography (SCXC) as well. To date, the structures of a series of thiolated metal nanoparticles with various sizes have been elucidated experimentally and theoretically [21] , [22] , [23] , [24] , [25] , [26] , [27] , [28] ; however, to the best of our knowledge, no structural isomerism in thiolated metal nanoparticles has been reported, albeit Au 24 (SCH 2 Ph- t Bu) 20 and Au 24 (SePh) 20 were revealed to have different Au 24 core structures [29] , [30] . In a strict sense, Au 24 (SCH 2 Ph- t Bu) 20 and Au 24 (SePh) 20 are not structural isomers, since their ligands are different. Thus, structural isomerism in thiolated nanoparticles remains a mystery. In the current work, using a modified synthesis method for Au 25 , we synthesize a nanocluster, whose composition is determined to be the same as that of the previously reported Au 38 (PET) 24 (refs 31 , 32 , 33 ) (PET, phenylethanethiolate), as evidenced by electrospray ionization mass spectrometry (ESI–MS) in combination with X-ray photoelectron spectroscopy (XPS) and thermogravimetric analysis (TGA). SCXC reveals that the structure of this nanocluster is different from that of the previously reported structure [24] . To differentiate the two structures, the previous Au 38 is denoted as Au 38Q and our nanocluster is denoted as Au 38T (where Q and T are the surname initial of the first author of the previous and current work, respectively). Au 38T and Au 38Q are therefore structural isomers and they represent the first pair of structural isomers in nanoparticles as revealed by SCXC, to the best of our knowledge. The two isomers exhibit distinctly different optical, stability and catalytic properties, and the less stable Au 38T can be irreversibly transformed to the more stable Au 38Q at 50 °C. Characterization Au 38T was synthesized using a modified one-pot method [34] and isolated using preparative thin-layer chromatography (PTLC) [35] , [36] . ESI–MS was employed to determine the exact molecular mass and formula of the novel nanoparticle (note: caesium acetate was added to form positively charged adducts). Three distinct peaks centred at m/z 10910.186, 7317.312 and 5522.217 were observed in the mass spectrum ( Fig. 1a ). The peaks at m/z 10910.186 and 5522.217 (almost half of 10910.186) can be readily assigned to [Au 38 (PET) 24 Cs] + (theoretical m/z value: 10910.658; deviation: 0.472) and [Au 38 (PET) 24 Cs 2 ] 2+ (theoretical m/z value: 5522.772; deviation: 0.555), respectively. The peak at m/z 7317.312 can be assigned to Au 26 (PET) 16 (theoretical m/z value: 7316.818; deviation: 0.494), which could be a fragment of Au 38 (PET) 24 , because the nanoparticles are monodisperse, as demonstrated by TLC, and it is also observed in the ESI spectrum of Au 38Q (see below). Based on the ESI–MS results, it is concluded that the as-prepared nanoparticle is neutral, and that its composition is Au 38 (PET) 24 , which is also corroborated by the TGA and XPS. TGA shows a weight loss of 30.39 wt% ( Fig. 1b ), corresponding to the theoretical loss of 30.55 wt% according to the formula. No other elements (including Cl, Br, N and Na) was detected by XPS ( Fig. 1c ), which excludes the possibility of existence of potential counterions such as Cl − , Br − , [N(C 8 H 17 ) 4 ] + and Na + ; thus, the as-prepared nanoparticle is neutral. Quantitative measurement reveals that the Au/S atomic ratio is 38.0:24.3 ( Supplementary Figs 3 and 4 ), in good agreement with the expected ratio (38.0:24.0) for the composition of Au 38 (PET) 24 . Thus, the formula is identical to that of the nanoparticle previously reported in ref. 31 ; however, the absorption spectrum of our nanoparticle distinctly differs from that of the previous nanoparticle. The ultraviolet–visible–near-infrared spectrum of the novel Au 38 (PET) 24 (abbreviated as Au 38T ) shows six absorption peaks at 505 nm (ɛ: 3.86 gcm l −1 ), 540 nm (ɛ: 3.22 gcm l −1 ), 610 nm (ɛ: 1.46 gcm l −1 ), 700 nm (ɛ: 0.69 gcm l −1 ), 880 nm and 1,090 nm ( Fig. 1d and Supplementary Fig. 2 ). The previous Au 38 (PET) 24 (abbreviated as Au 38Q ) shows six absorption peaks centred at 480 nm (ɛ: 4.62 gcm l −1 ), 520 nm (ɛ: 3.72 gcm l −1 ), 570 nm (ɛ: 2.86 gcm l −1 ), 627 nm (ɛ: 2.59 gcm l −1 ), 740 nm (ɛ: 0.58 gcm l −1 ) and 1,035 nm ( Fig. 1d and Supplementary Fig.1 ). TLC also indicates that they are not the same nanoparticle ( Fig. 1d , inset). Indeed, they are a pair of structural isomers (vide infra). 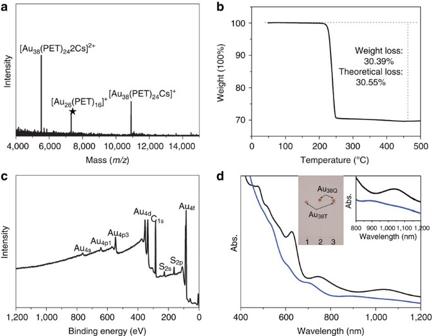Figure 1: Characteriztion of Au38T. (a) ESI mass spectrum of the Au38T. (b) TGA of Au38T. (c) XPS spectrum of Au38T. (d) Ultraviolet–visible–near-infrared absorption spectra of Au38T(blue) and Au38Q(black) in toluene (measurement temperature: 0 °C). Insets are the photo of thin-layer chromatography, and enlarged absorption spectra in the range from 800 to 1,200 nm of Au38Tand Au38Q. Figure 1: Characteriztion of Au 38T . ( a ) ESI mass spectrum of the Au 38T . ( b ) TGA of Au 38T . ( c ) XPS spectrum of Au 38T . ( d ) Ultraviolet–visible–near-infrared absorption spectra of Au 38T (blue) and Au 38Q (black) in toluene (measurement temperature: 0 °C). Insets are the photo of thin-layer chromatography, and enlarged absorption spectra in the range from 800 to 1,200 nm of Au 38T and Au 38Q . Full size image Atomic structure The structure of the previous Au 38Q was determined by SCXC and it has a core-shell structure consisting of a face-fused bi-icosahedral Au 23 core, which is capped by a second shell composed of the remaining 15 gold atoms ( Fig. 2f ). To confirm that our nanoparticle (Au 38T ) is an isomer of Au 38Q , we grew high-quality single crystals and successfully elucidated the structure via SCXC. Briefly, the new structure of Au 38T is composed of one Au 23 core and one mixed capping layer of thiolate ligands and gold–thiolate complex units. The Au 23 core consists of one icosahedral Au 13 and one Au 10 unit, and the mixed surface layer contains two Au 3 (SR) 4 staple units, three Au 2 (SR) 3 staple units, three Au 1 (SR) 2 staple units and one bridging thiolate SR ligand. The anatomy of the Au 38T structure starts with the central Au 23 core ( Fig. 2b ), which can be viewed as one Au 12 cap and one Au 13 icosahedron ( Fig. 2a ) fused together via sharing two gold atoms ( Fig. 2b , dark green gold atoms), which is in distinct contrast with the case of Au 38Q ; for the latter, the two Au 13 icosahedra are fused together via sharing a face (three gold atoms) to form a bi-icosahedral Au 23 core. The Au 12 cap is composed of three tetrahedra and the Au–Au bond lengths in each tetrahedron range from 2.71 to 2.88 Å. In the Au 13 icosahedron, the Au–Au bond lengths between the central atom and the shell Au atoms (except for the two shared gold atoms) vary from 2.71 to 2.82 Å. The bond lengths between the two shared gold atoms and the central atom of Au 13 icosahedron are 2.77 and 2.78 Å, respectively. The different Au 23 core in Au 38T (in contrast to the biicosahedral Au 23 core of Au 38Q ) leads to various surface-binding structures. The Au 23 core in our case was capped by two Au 3 (SR) 4 units and two Au(SR) 2 units, and the average Au–S bond lengths/Au–S–Au bond angles were 2.33 Å/96.47° and 2.32 Å/94.43° in the Au 3 (SR) 4 and Au(SR) 2 staple units, respectively ( Fig. 2c ). Interestingly, in addition to the two Au 3 (SR) 4 units and two Au(SR) 2 units, one bridging thiolate (SR) is also found to link the Au 13 icosahedron and the Au 12 cap ( Fig. 2c , the sulfur atom is marked in red), the two Au–S bond lengths are 2.33 and 2.30 Å, respectively, and the Au–S–Au bond angle is 92.66°. It is noteworthy that in Au 38Q , the Au 23 core was protected by six Au 2 (SR) 3 and three Au(SR) 2 staple units; no comparable Au 3 (SR) 4 staple units and bridging thiolate (SR) was observed. The Au 13 icosahedron in Au 38T is exclusively capped by two Au 2 (SR) 3 staple units (the average Au–S bond lengths in the Au 2 (SR) 3 staple units are 2.35 and 2.34 Å, respectively, and the average Au–S–Au bond angles in the Au 2 (SR) 3 staple units are 92.20° and 90.33°, respectively) and the Au 12 cap is capped by one Au 2 (SR) 3 staple unit (the average Au–S bond length is 2.33 Å and the average Au–S–Au bond angle is 97.03°). In addition, the Au 12 cap is also capped by one Au(SR) 2 staple unit, and the average Au–S bond length/Au–S–Au bond angle are 2.33 Å and 99.91° ( Fig. 2d ). The structure resolved by X-ray diffraction was further analysed by computations: the simulated ultraviolet–visible–near-infrared spectrum is close to the experimental one ( Fig. 3 ). 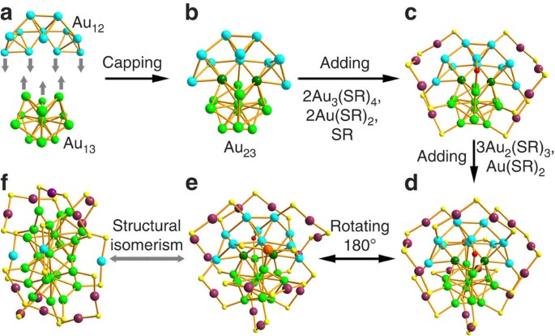Figure 2: Structures of Au38Tand Au38Q. (a) Anatomy of the Au23core, which consists of a Au12cap unit and Au13icosahedral unit. (b) Au23core, which is constructed by one Au12unit and one Au13unit sharing two gold atoms. (c) Two Au3(SR)4, two Au(SR)2and one SR linking the Au12cap and Au13icosahedron. (d) Three Au2(SR)3and one Au(SR)2protecting the Au23core. (e) Back view of Au38T. (f) The Au38Qstructure. Figure 2: Structures of Au 38T and Au 38Q . ( a ) Anatomy of the Au 23 core, which consists of a Au 12 cap unit and Au 13 icosahedral unit. ( b ) Au 23 core, which is constructed by one Au 12 unit and one Au 13 unit sharing two gold atoms. ( c ) Two Au 3 (SR) 4 , two Au(SR) 2 and one SR linking the Au 12 cap and Au 13 icosahedron. ( d ) Three Au 2 (SR) 3 and one Au(SR) 2 protecting the Au 23 core. ( e ) Back view of Au 38T . ( f ) The Au 38Q structure. 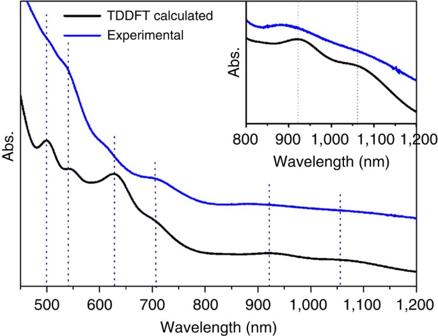Figure 3: Comparison of ultraviolet–visible–near-infrared absorption spectra of Au38T. Blue: experimental; black: calculated by time-dependent density function (TDDFT) method. Inset is the enlarged spectra in the range from 800 to 1,200 nm. Full size image Figure 3: Comparison of ultraviolet–visible–near-infrared absorption spectra of Au 38T . Blue: experimental; black: calculated by time-dependent density function (TDDFT) method. Inset is the enlarged spectra in the range from 800 to 1,200 nm. Full size image As discussed above, the structure of Au 38T is remarkably different from that of Au 38Q and the main differences between the two structures lie in the type of Au 23 core and the surface capping mode of the Au 23 core. Au 38T and Au 38Q have an identical composition but completely different structures; thus, they are literally a pair of structural isomers. Notably, the structure of Au 38T reported in this work is novel and also differs from those theoretical structures predicted by Hakkinen et al . [37] , Tsukuda and colleagues [38] , Jiang et al . [39] and Zeng and colleagues [40] , among others. Transformation Au 38T exhibits relatively high stability at low temperatures, as no obvious spectral changes was detected when a solution of Au 38T was stored at −10 °C for as long as 1 month in toluene ( Fig. 4a ). However, the absorption spectrum of Au 38T gradually changed to that of Au 38Q at 50 °C in toluene ( Fig. 4b ), which indicates that Au 38T can transform to Au 38Q at elevated temperatures. TLC and ESI–MS further support this transformation ( Fig. 4b (inset) and Fig. 4c ). However, the reverse transformation (that is, from Au 38Q to Au 38T ) was not successful under various investigated conditions. These results indicate that Au 38T is less stable than Au 38Q , and that Au 38T can only be irreversibly transformed to Au 38Q . The reason for why the relatively unstable Au 38T is formed rather than the stable Au 38Q during the synthesis is probably because the former is kinetically favourable in our reaction conditions, similar to some previous reports [41] , [42] . 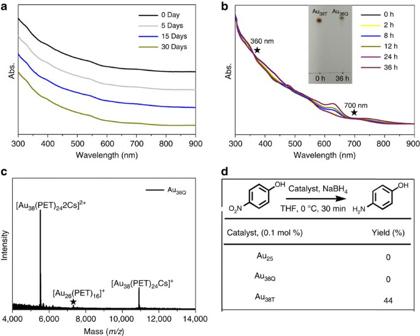Figure 4: Difference in stability and catalysis between Au38Tand Au38Q. (a) Time-dependent ultraviolet–visible–near-infrared absorption spectra of Au38Tat −10 °C in toluene. (b) Ultraviolet–visible–near-infrared absorption spectral transformation at 50 °C in toluene (the isosbestic points are at 360 and 700 nm). Inset: thin-layer chromatography of Au38Tbefore and after the transformation. (c) ESI mass spectrum of the transformed product. (d) Catalytic activities of Au25, Au38Tand Au38Q. Figure 4: Difference in stability and catalysis between Au 38T and Au 38Q . ( a ) Time-dependent ultraviolet–visible–near-infrared absorption spectra of Au 38T at −10 °C in toluene. ( b ) Ultraviolet–visible–near-infrared absorption spectral transformation at 50 °C in toluene (the isosbestic points are at 360 and 700 nm). Inset: thin-layer chromatography of Au 38T before and after the transformation. ( c ) ESI mass spectrum of the transformed product. ( d ) Catalytic activities of Au 25 , Au 38T and Au 38Q . Full size image Catalysis Au 38T exhibits remarkably higher catalytic activity than Au 38Q at low temperature (for example, 0 °C) in reduction reactions. For example, 4-nitrophenol can be reduced to 4-aminophenol in 44% yield with 0.1 mol% Au 38T catalyst in half an hour, whereas no reduction occurred when Au 25 (PET) 18 − TOA + (Au 25 for short, TOA + : tetra- n -octylammonium) or Au 38Q was used as the catalyst ( Fig. 4d and Supplementary Fig. 5 ) under the same reaction conditions. It is noteworthy that in other cases, Au 25 was reported to exhibit good catalytic reduction activity [43] , [44] . The high catalytic activity of Au 38T may be due to its surface being not as densely protected as the surfaces of Au 25 and Au 38Q ; further investigation is underway. A previous work [44] implied that the catalytic properties of gold nanoclusters are not only size dependent but also structure sensitive. However, the structure dependence of catalytic properties was unclear at that time, because the ligands were different in Au 44 (PET) 32 and Au 44 (TBBT) 28 (TBBT: 4-tert-butylbenzenethiolate), and the ligand effect should be considered. Herein, it is unambiguously demonstrated that the structure effect indeed exists, because Au 38T and Au 38Q exhibit remarkably different catalytic performance. Au 38T is relatively robust and can retain its ultraviolet–visible–near-infrared spectrum even after 18 catalytic cycles ( Supplementary Fig. 6 ). It is noteworthy that the gradual decrease in the yield is primarily due to the unavoidable mass loss of the catalyst during the isolation by column chromatography. However, after 21 cycles, the catalyst transformed to more stable Au 38Q demonstrated by the ultraviolet–visible–near-infrared spectra and accordingly the loss of catalytic activity (see Supplementary Table 1 ). The high catalytic activity at low temperatures indicates the potential application of Au 38T in some catalytic processes. In summary, we have discovered a pair of structural isomers Au 38T and Au 38Q , which were identified using ESI–MS, TGA, XPS and SCXC. Although both species have the same composition (that is, Au 38 (PET) 24 ), they have distinctly different structures, which results in differences in their optical and catalytic properties, as well as structural stability. The less stable Au 38T can be irreversibly transformed to the more stable Au 38Q at high temperatures. The structure of Au 38T is very interesting: it is composed of a Au 23 core (fused by one Au 13 icosahedron and one Au 12 cap by sharing two atoms) and a mixed layer of thiolate ligands and gold–thiolate complex units for surface protection. This structure is unique (that is, not found in other reported gold nanoclusters). In particular, the diversity of staple units and the bridging thiolate found in Au 38T provide a new direction for structural studies of metal nanoclusters. The significance and novelty of this work are as follows. (i) A novel synthesis method is developed, with which a novel gold nanoparticle is readily synthesized, and the composition of the as-prepared nanoparticle is precisely determined using ESI–MS in conjunction with XPS and TGA. (ii) The structure of Au 38T is resolved using SCXC and the unique structural features provide important implications for nanocluster structural studies. (iii) Significantly, structural isomerism is observed in nanoparticles for the first time. (iv) The distinctly different properties (in particular the catalytic properties) of the two structural isomers indicate a structure–property correlation and this will have important implications for future catalytic studies. It is expected that our work may motivate more studies on structural isomerism and structure–property correlations in nanoscale or even larger scale materials. Reagents All chemicals and reagents are commercially available and were used as received. Tetraoctylammonium bromide (TOAB, 98.0%) and 4-nitrophenol (99.0%) were obtained from Aladdin; 2-phenylethanethiol (PhC 2 H 4 SH, 99.0%) was purchased from Sigma-Aldrich; Au 38Q and Au 25 (PET) 18 − TOA + were synthesized following reported methods [31] , [34] . Synthesis Au 38T was synthesized using a modified one-pot method and separated using PTLC. Briefly, HAuCl 4 ·4H 2 O (0.20 g, 0.48 mmol) was mixed with 1.03 equivalents of TOAB (0.27 g, 0.49 mmol) in CH 2 Cl 2 (40 ml). Then, 9 equivalents of phenylethanethiol (0.61 ml, 4.50 mmol) were added to this solution and the solution was stirred for ∼ 2 h until it became colourless. To this solution, 5.3 equivalents of NaBH 4 (0.11 g, 2.80 mmol) in cold water (5 ml) was added in one shot under vigorous stirring and the reaction was allowed to proceed under constant stirring for 6 h. CH 2 Cl 2 was removed via rotary evaporation at 20 °C to isolate the crude product. For purification, the crude product was extracted with a small amount of tetrahydrofuran (THF) and washed with ice water three times and with CH 3 OH two times; during this procedure, traces of inorganic salt, excess TOAB and phenylethanethiol were thoroughly removed. Next, the as-obtained crude products were separated using PTLC (dichloromethane: petroleum ether=3:4) and finally the target product was isolated from the reddish brown band of PTLC after extraction with CH 2 Cl 2 , with a yield of 5%. Characterization The ultraviolet–visible–near-infrared absorption spectrum was measured on a UV-3600 spectrophotometer (Shimadzu, Japan) at room temperature. TGA analysis was conducted under a N 2 atmosphere ( ∼ 3 mg sample used, flow rate ∼ 50 ml min −1 ) on a TG/DTA 6300 analyzer (Seiko Instruments, Inc.) and the heating rate was 10 °C min −1 . XPS measurements were performed on an ESCALAB 250Xi XPS spectrometer (Thermo Scientific, USA), using a monochromated Al Kα source and equipped with an Ar + ion sputtering gun. All binding energies were calibrated using the C (1 s) carbon peak (284.8 eV). ESI–MS data were acquired on a Waters Q-TOF mass spectrometer equipped with a Z-spray source. The sample was dissolved in toluene ( ∼ 1 mg ml −1 ) and diluted 1:1 in dry ethanol (5 mM CsOAc). The sample was directly infused at 5 μl min −1 . The source temperature was fixed at 70 °C. The spray voltage was set at 2.20 kV and the cone voltage was set at 60 V. Single-crystal growth and analysis Black crystals were formed from a CH 2 Cl 2 /hexane solution of the nanoclusters at 4 °C after 5 days. The diffraction data for Au 38 (PET) 24 were collected at 173 K on a Bruker APEX DUO X-ray diffractometer using Cu Kα radiation ( λ =1.54184 Å). Theoretical methods All calculations were performed using density functional theory with the pure functional Perdew-Burke-Ernzerhof [45] , [46] and the all electron basis set 6–31 g ( d , p ) for H, S, pseudopotential basis set LANL2DZ for Au, as implemented in the Gaussian 09 program package [47] . Time-dependent density functional calculations [48] were performed to reproduce the experimental ultraviolet–visible spectrum and –R group was replaced by –H to minimize computational work [31] . The Gaussian half-width at half-height of 0.15 eV in the Multiwfn software [49] was used to simulate the ultraviolet–visible spectrum. General procedure for the catalyses 4-Nitrophenol (69.50 mg, 0.500 mmol), Au 38Q , Au 25 or Au 38T (0.100 mol%, not adsorbed on a support or calcined) and THF (5 ml) were mixed in a reaction tube at 0 °C. The mixture was stirred at this temperature for 5 min. NaBH 4 (189.00 mg, 5.000 mmol) dissolved in 1.0 ml of H 2 O was added slowly to the mixture. After stirring at 0 °C for 30 min, a large amount of water was added to quench the reaction. The mixture was extracted with dichloromethane twice (2 × 10 ml) and then the organic layers were collected and concentrated. The reduction product (4-aminophenol) was purified by column chromatography on silica gel, with ethyl acetate and petroleum ether (ethyl acetate/petroleum ether=1/1) as the eluant. General procedure for the recovery of Au 38T When the reduction was completed, the reaction mixture was quenched with water. Au 38T and other organic compounds were extracted with dichloromethane. The extract was collected and concentrated. After the other organic compounds were isolated by column chromatography with ethyl acetate and petroleum ether, Au 38T was recovered using dichloromethane as the eluant. The dichloromethane was evaporated under reduced pressure and then Au 38T was re-used in the next cycle without further treatment. Accession codes: The X-ray crystallographic coordinates for structures reported in this study (see Supplementary Table 2 and Supplementary Data 1 ) have been deposited at the Cambridge Crystallographic Data Centre (CCDC), under deposition number CCDC 1423153. These data can be obtained free of charge from The Cambridge Crystallographic Data Centre via www.ccdc.cam.ac.uk/data_request/cif . How to cite this article: Tian, S. et al . Structural isomerism in gold nanoparticles revealed by X-ray crystallography. Nat. Commun. 6:8667 doi: 10.1038/ncomms9667 (2015).